Nanotwin-assisted grain growth in nanocrystalline gold films under cyclic loading Under mechanical loading, nanocrystalline metals show unique behaviour, among the most common of which are high strength, mechanically induced grain growth and twin formation. However, mechanically induced grain growth is seldom correlated with twins. Here we report a clear relationship between grain growth and nanoscale twins in 20-nm-thick gold films with a grain size of ~19 nm under cyclic loading based on atomic-scale observations and analyses. We find that the formation of nanotwins is an effective way to assist grain coarsening, following a fundamental process that the mutual formation of nanotwins in two neighbouring grains changes the local grain orientation and dissociates the grain boundary into new segments, which become more mobile. The proposed mechanism of nanotwin-assisted grain growth may have important implications for understanding the interface-mediated mechanisms of cyclic plastic deformation and for the interface engineering design of nanostructured metals with both high strength and good fatigue resistance. Although a grain boundary (GB), as an effective barrier to dislocation motion, plays a key role in enhancing yield strength of polycrystalline metals through reducing grain size down to nanometre scales, GBs in nano-grained metals usually become so unstable that grain growth characterized by GB migration/grain coarsening always occurs. Grain growth is most commonly associated with thermally activated GB migration [1] , [2] , but it was also observed in nanocrystalline (nc) copper deformed at liquid-nitrogen temperature [3] , indicating that the grain growth in nc metals could be induced mechanically. Furthermore, Rupert et al. [4] have experimentally uncovered the shear-stress-driven GB migration behaviour in the aluminium film using the specimens smartly designed with stress and strain concentrators. Until now, the grain growth has been observed under various loading modes including tension [5] , [6] , compression [7] , nanoindentation [3] , [8] and cyclic deformation [9] , [10] . Several mechanisms are currently correlated to mechanically induced grain growth such as grain rotation and agglomeration [11] , [12] , GB migration [4] , [13] , cooperative mechanism [11] , [14] , [15] , and so on. It is suggested that the grain rotation is a significant factor only for very small grains and at very high temperatures [1] , and the growth mechanism is associated with gradual GB dissociation caused by dislocation motion [15] , [16] . For GB migration, the motion of a low-angle GB (LAGB) is generally related to the collective motion of the individual dislocations in these boundaries [17] , [18] , [19] , [20] , while the migration of a high-angle GB (HAGB) is mainly described by the shuffling model [21] , the DSC (displacement shift complete) model [22] , [23] , [24] and the shear coupling models [13] , [25] , [26] . In the DSC model, the HAGB migration is attributed to the motion of the secondary GB dislocations, which result in a combined GB migration and sliding [27] . Cahn et al. [13] , [25] have recently proposed a unified approach to the GB motion in the shear coupling mode. Furthermore, a more generalized formulation [28] was proposed to describe the shear-migration coupling of ordinary GBs with non-coincidence relationships and irrational habit planes. Upon plastic deformation of the nc fcc-structured metal, Shockley partial dislocations (PDs) are usually emitted from GBs [29] , leading to frequent twin nucleation. Besides, molecular dynamics simulation [30] and experimental observations [31] , [32] suggest that twins can form by GB motion or dissociation. These twin-related GB activities may give rise to questions whether the GB migration is related to nanotwins. If so, the question arises how these GBs migrate through formation of nanotwins and how the nanograins become coarsened. In this communication we show that grain growth of 20-nm-thick gold films with a grain size of ~19 nm under fatigue loading has a close relationship to nanotwins. The twin formation in nano-grained gold films is an effective way to gradually change the local grain orientation from the high-angle misorientations to the low-angle misorientations. Frequent formation of twins can lead to the consequent dissociation of GBs and accelerated GB migration, which remarkably promote grain growth in the nano-grained gold films subjected to fatigue loading. Microstructures of the gold films Transmission electron microscopy (TEM) bright-field images on both plan-view ( Fig. 1a ) and cross-sectional view ( Fig. 1b ) indicate that the as-deposited film has a columnar grain structure with an in-plane grain size of 19.0±7.6 nm. Here twin boundaries (TBs) were ignored in the determination of the grain size. Some of the grains have growth twins ( Fig. 1b ). X-ray diffraction θ–2θ scans (see inset in Fig. 1a ) reveal that the film has a strong (111) out-of-plane texture. 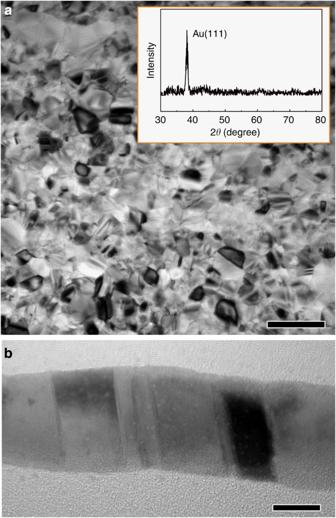Figure 1: Microstructure and texture. (a) Plan-view and (b) cross-sectional view bright-field TEM images of the as-deposited gold film, showing a columnar grain structure with some growth twins. Inset is XRDθ–2θscanning result, revealing a strong (111) out-of-plane texture. Scale bars: (a) 50 nm, (b) 10 nm. Figure 1: Microstructure and texture. ( a ) Plan-view and ( b ) cross-sectional view bright-field TEM images of the as-deposited gold film, showing a columnar grain structure with some growth twins. Inset is XRD θ –2 θ scanning result, revealing a strong (111) out-of-plane texture. Scale bars: ( a ) 50 nm, ( b ) 10 nm. Full size image We firstly examined the 20-nm-thick gold film sample, in which fatigue damage happened within 10 6 cycles under a total strain range of 1.41%. Such a strain range is expected to cause a high stress range [33] . Features of fatigue damage in the gold film ( Fig. 2a ) mainly exhibit multiple cracks without any bulk-like fatigue extrusions/intrusions induced by cyclic strain localization [34] . Then, we carefully checked the cyclically deformed regions far away from and near the cracks, as shown in Fig. 2b,c , respectively. Obvious grain growth was found in both regions. The mean grain size of the fatigued sample has increased to 41.3±15.4 nm compared with that (19.0±7.6 nm) of the as-deposited sample (see Fig. 2d ), and the grain size distribution broadens as the grain size increases. Especially, there is no appreciable difference in the extent of grain coarsening between the two regions, implying that the grain growth in the present nano-grained film is locally uniform. 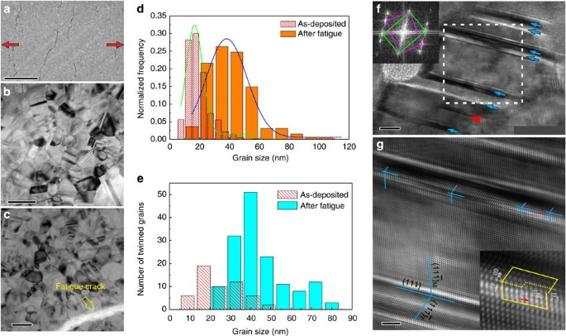Figure 2: Fatigue damage behaviour and quantitative characterization. (a) Scanning electron microscopy (SEM) observation of damage morphology in the 20-nm-thick gold film after fatigue loading. (b,c) TEM images for places far away from the cracks and near the cracks, respectively. Statistical distributions of (d) normalized frequency and (e) the number of twinned grains with grain size in as-deposited and fatigued samples. (f)HRTEM image of a typical large grain with parallel multi-twins, showing seven twin planes indicated by arrows. The red arrow indicates a stacking fault. The inset is the fast Fourier transformations of one twin. (g) A high magnification of nanotwins in dash-squared region in (f). TB steps show imperfect twin boundaries. The inset is the Frank circuit with a closure failure. Scale bars: (a) 2 μm, (b,c) 50 nm, (f) 5 nm, (g) 2 nm. Figure 2: Fatigue damage behaviour and quantitative characterization. ( a ) Scanning electron microscopy (SEM) observation of damage morphology in the 20-nm-thick gold film after fatigue loading. ( b , c ) TEM images for places far away from the cracks and near the cracks, respectively. Statistical distributions of ( d ) normalized frequency and ( e ) the number of twinned grains with grain size in as-deposited and fatigued samples. ( f ) HRTEM image of a typical large grain with parallel multi-twins, showing seven twin planes indicated by arrows. The red arrow indicates a stacking fault. The inset is the fast Fourier transformations of one twin. ( g ) A high magnification of nanotwins in dash-squared region in ( f ). TB steps show imperfect twin boundaries. The inset is the Frank circuit with a closure failure . Scale bars: ( a ) 2 μm, ( b , c ) 50 nm, ( f ) 5 nm, ( g ) 2 nm. Full size image Coarsening of twinned grains We surprisingly found that the coarsened grains had a close correlation with twin formation. After examining ~740 grains in the fatigued samples and in the as-deposited ones respectively, we noticed that the fraction of nanotwins evidently increased and many coarsened grains contained multiple nanotwins in the fatigued samples. The distribution range of the size of twinned grains after cyclic deformation has shifted from the original range (5–50 nm) to that with larger grains (20–80 nm). Meanwhile, the number of the twinned grains also greatly increased ( Fig. 2e ). Figure 2f shows a typical multi-twinned grain with an average twin spacing of 5 nm. The TBs in the grain are generally imperfect, as characterized by a high-resolution transmission electron microscopy (HRTEM) image ( Fig. 2g ). Here the Frank circuit (see inset in Fig. 2g ) with a closure failure of , which is the projected vector of Shockley PD on the plane. A number of HRTEM observations further show the appearance of nanotwins, stacking faults and multi-twinned grains (see Supplementary Figs S1–3 ). At present, it is not definitely proven that these nanotwins are deformation twins rather than growth twins. Nanotwin-assisted GB dissociation Through the following two examples of the fatigued samples, we will uncover a mechanism for the observed grain growth, essentially being the process of nanotwin-assisted GB dissociation and local grain coarsening. The first example ( Fig. 3a ) shows an HRTEM image of two large grains ( G1 and G2 ) with typical multi-twins (note that the lower right grain labelled by G1 is partly shown but the un-imaged part of the GB was schematically marked by asterisks). 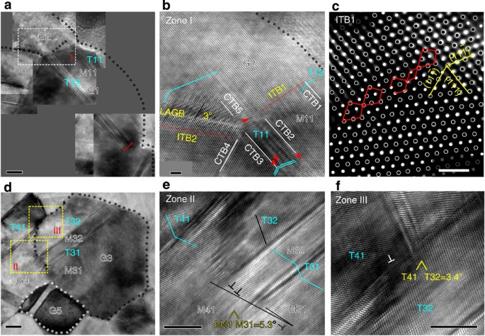Figure 3: GB dissociation induced by twin formation. (a,d) HRTEM images of two typical examples for large grains (G1 and G2 for example 1, G3 and G4 for example 2) with parallel multi-twins in the fatigued samples. (b,c) and (e,f) The corresponding details of the microstructures for examples 1 and 2, respectively. Asterisks indicate GBs.TandMare abbreviation of twin and matrix, respectively. Red arrows indicate stacking faults. In (a),T11terminates in the grain, and stacking faults at the tip of theT11are indicated by arrows. (b) A close observation of zone I ina. Red dashed lines indicate the incoherent TB (ITB). (c) Boundary structure ofITB1. (e) A high magnification of zone II in (d), the twinning relationship is marked by the solid line.G4(M41)andG3(M31)have a small misorientation of 5.3°. Three perfect dislocations are indicated by a symbol ‘⊥’. (f) A close examination of zone III ind,T41andT32has a small misorientation of 3.4°. A perfect dislocation is indicated by a symbol ‘⊥’. The misorientation angles are determined by the angle between {111} planes, which is labelled by the black straight lines, as shown inbande. Scale bars: (a,d–f) 5 nm, (b,c) 1 nm. Figure 3b reveals that the misorientation between G1 and the upper left grain ( G2 ) is 60°, as a HAGB. The 2-nm-wide twin lamella ( T11 ) terminated in G1 and changed the local orientation of G1 to the same orientation as G2 (similarly T12 and G2) . As a result, some parts of G1 were transformed into G2 through such multiple formation of nanotwins, which made the boundary between G1 and G2 dissociate gradually. According to Fig. 3c , we know that the remaining part of the GB is a Σ3{112} incoherent TB, which is the relaxed 9R boundary structure, as reported in the literature [35] , [36] . Obviously, such frequent formation of nanotwins gradually changed the orientation of the grain into that close to the orientation of the neighbouring grain. Figure 3: GB dissociation induced by twin formation. ( a , d ) HRTEM images of two typical examples for large grains (G1 and G2 for example 1, G3 and G4 for example 2) with parallel multi-twins in the fatigued samples. ( b , c ) and ( e , f ) The corresponding details of the microstructures for examples 1 and 2, respectively. Asterisks indicate GBs. T and M are abbreviation of twin and matrix, respectively. Red arrows indicate stacking faults. In ( a ), T11 terminates in the grain, and stacking faults at the tip of the T11 are indicated by arrows. ( b ) A close observation of zone I in a . Red dashed lines indicate the incoherent TB (ITB). ( c ) Boundary structure of ITB1 . ( e ) A high magnification of zone II in ( d ), the twinning relationship is marked by the solid line. G4(M41) and G3(M31) have a small misorientation of 5.3°. Three perfect dislocations are indicated by a symbol ‘ ⊥ ’. ( f ) A close examination of zone III in d , T41 and T32 has a small misorientation of 3.4°. A perfect dislocation is indicated by a symbol ‘ ⊥ ’. The misorientation angles are determined by the angle between {111} planes, which is labelled by the black straight lines, as shown in b and e . Scale bars: ( a , d – f ) 5 nm, ( b , c ) 1 nm. Full size image Another example is presented by the HRTEM observation on two larger grains ( G3 and G4 ) and a smaller grain ( G5 ) (see Fig. 3d ). G3 and G4 had a LAGB with a misorientation of 5.3° ( Fig. 3e ). When nanotwins T31 and T32 formed in G3 , they impinged on the LAGB and transformed local parts of the LAGB into several boundary segments with a larger angle, which are energetically more favourable than the LAGB for GB migration [8] , [15] , [37] . The local orientation of a nanotwin T41 in G4 keeps the orientation close to that of T32 in G3 (only 3.4°), and a perfect dislocation on such a LAGB was also found in Fig. 3f . Our observations mainly reveal that twin formation may play an important role in the grain growth, but such a twin-assisted mechanism does not exclude other mechanisms for grain growth [4] , [11] , [25] , [38] , such as some full/partial dislocations are likely to be involved in the dissociation of the GB, having no relationship with twin formation and the surface/boundary effects may also not be neglected. In spite of this, one would like to know how large are the driving forces of twin nucleation and grain growth, and what is the relationship between twin formation and grain growth under cyclic loading? First, we calculate the driving force for twin nucleation, which reveals that PDs in gold would be activated preferentially as the grain size deceases down to ~20 nm (see Supplementary Discussion and Supplementary Fig. 4 ). Thus, PDs to form a twin would be present in some nanograins in the 20-nm-thick gold film with grains ranging from 5–50 nm. Second, diffusion mechanisms like Coble creep and GB sliding are not the necessary conditions for the grain growth of very small grains [3] , [38] . Grain growth is generally driven by the reduction in the overall free energy [5] , [27] , traditionally including a decrease in stored deformation energy, elastic strain energy, GB energy or surface energy [27] . Here we firstly consider the traditional driving force for grain growth and then the mechanical stress. (a) An excess density of defects (for example, dislocations) is a powerful source of a driving force [27] . Here no dislocation networks are observed in both the as-deposited and the as-deformed samples, so the contribution of the stored deformation energy could be neglected. (b) The elastic driving force P can be simply given by the difference in the stored elastic energy density of the two grains [27] where τ is the elastic stress ~10 2 MPa. E 1 and E 2 are elastic moduli of neighbouring grains ~10 5 MPa, respectively. Thus, the diving force is about three orders of magnitude lower than the elastic stress. (c) The reduction in the GB energy and the surface energy also promotes the grain growth. These two types of driving forces dominate the grain growth at elevated temperature in metal films. Thus, we conducted annealing treatment at 250 °C for ~10 h in vacuum to see how the two factors affect the grain growth. Here the annealing time was approximately equal to the fatigue testing time. Furthermore, we calculate and compare the creep rate under the stress-driven condition and the thermally driven condition according to the Coble creep equation [39] . where A is a constant, σ is the stress, d is the average grain size, H b is the activation energy ( H b =173.4 kJ mol −1 ) [27] , R is the gas constant and T is the temperature. The calculation results presented in Table 1 indicate that is much larger for the annealed sample, even if an underestimated stress is chosen. However, the annealed gold film does not show a more noticeable predominance in grain growth, instead, the average grain size of the annealed sample is smaller than that of the fatigued sample, as shown in Figs 1a and 4 . This confirms that the mechanical stress plays an important role in promoting grain growth. Table 1 A comparison of creep rates of the gold film under fatigue loading and annealing treatment. 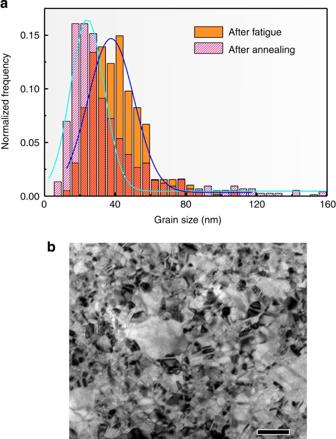Figure 4: Statistic of grain size and observation. (a) Statistical distribution of grain size in fatigued and annealed gold films. The average grain size of the annealed sample is smaller than that of the fatigued sample. (b) Plan-view TEM image of microstructures of the annealed 20-nm-thick gold film. Scale bar: 100 nm. Full size table Figure 4: Statistic of grain size and observation. ( a ) Statistical distribution of grain size in fatigued and annealed gold films. The average grain size of the annealed sample is smaller than that of the fatigued sample. ( b ) Plan-view TEM image of microstructures of the annealed 20-nm-thick gold film. Scale bar: 100 nm. Full size image Third, we estimated the driving force for mechanically driven grain growth based on the presently available models [38] . The comparison of the driving force between twin formation and grain growth (see Supplementary Discussion and Supplementary Table S1 ) indicates that their driving forces are comparable. Whether the twin formation or grain growth happens may depend on the applied stress. It is believed that the twin formation and grain growth would occur simultaneously because of the larger applied stress in the gold film. Alternatively, even if the grain growth happened prior to the twin formation at the first-cycle loading, the nanotwins formed in the subsequent-cycle loading would immediately participate in the GB dissociation and grain coarsening, as observed in Figs 2 and 3 . As the cyclic stress in the film varies periodically from the maximum to the minimum, sometimes it would get smaller than both stresses for twin formation and grain growth, leading to the repeated growth process starting from twinned grains. Especially, the pre-existing growth nanotwins may also be involved in the GB dissociation at the first onset of the grain growth in the first-cycle loading. Thus, whether the nanotwins formed before or after the onset of grain growth in the first-cycle loading, they always assisted GB dissociation with the accumulation of cyclic loading. Based on our atomic-scale observations, the nanotwin-assisted grain growth mechanism in the cyclically deformed nc gold films can be illustrated schematically in Fig. 5 . The cyclic loading sustains the successive formation of nanotwins in the one/two grains, which frequently impinge on the GB, leading to the local dissociation of the GB ( Fig. 5a–d ). The formation of nanotwins may lead to the fact that some local parts of the HAGB are transformed into several new LAGB segments. Generally, the LAGB segments are several nanometres in length with one or two dislocations, as observed in Fig. 3e,f . These very limited dislocations could be either removed by reaching the nearby boundaries [38] , [40] or dissociated to glide into a coherent TB [29] , [41] . Besides, the undissociated segments of the HAGB would become much easier to move than the whole HAGB under the mechanical stress ( Fig. 5e ), because the velocity of the GB motion is inversely proportional to the size of the moving unit [20] , [42] . All these twin-related activities promote two grains to gradually coalesce into one grain with multiple twins ( Fig. 5f ). A similar grain growth process would occur in the grains with LAGBs. The nanoscale grain size smaller than 10–20 nm results in the fact that the PDs are more prevalent [29] , while twin formation sustained by cyclically loading–unloading gradually depletes the whole grain through continuous formation of twins inside the grains. In what follows, we will consider a general case where the orientation relation between the two grains fits such local grain coalescence. 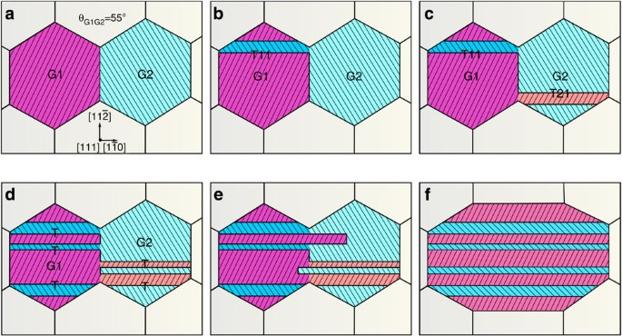Figure 5: Schematic illustration of nanotwin-assisted grain growth mechanism. (a) Two nanograins (G1andG2) in the gold film with the [111] out-of-plane texture before cyclic deformation. (b,c) Twin formation inG1andG2produces nanotwinsT11andT21respectively, leading to local dissociation of GB. Orientations ofT11andT21are close to that ofG2andG1, respectively. (d) Successive twin formation within two grains further splits the GB. (e) Undissociated segments of GB move into the neighbor grain. (f) Coupled with the GB motion, two grains finally coalesce into one grain with multiple twins. Figure 5: Schematic illustration of nanotwin-assisted grain growth mechanism. ( a ) Two nanograins ( G1 and G2 ) in the gold film with the [111] out-of-plane texture before cyclic deformation. ( b , c ) Twin formation in G1 and G2 produces nanotwins T11 and T21 respectively, leading to local dissociation of GB. Orientations of T11 and T21 are close to that of G2 and G1 , respectively. ( d ) Successive twin formation within two grains further splits the GB. ( e ) Undissociated segments of GB move into the neighbor grain. ( f ) Coupled with the GB motion, two grains finally coalesce into one grain with multiple twins. Full size image We can simply describe the twin orientation relationship as 180°<111> considering the high crystal symmetry in the fcc crystal [43] , [44] , and the corresponding matrices Γ twin are listed as follows: For a grain G with an orientation of M G, the orientation of the twin T in G can be described by M twin = Γ twin · M G . The misorientation between any two orientations ( M A and M B ) can be expressed as Γ mis = M B ·inv( M A ). We can derive the axis and its corresponding rotation angle (also called misorientation angle) from the matrix Γ mis (more details in ref. 45 ). Then, 24 symmetry operators (for cubic symmetry) are used to get the smallest rotation angle among all symmetrically equivalent misorientation angles. Since the angle for the transition from low to high angle boundaries is typically taken as between 10° and 15°, 10° is chosen as a critical angle misorientation ( θ c ) below which the two coalesced grains are locally regarded as one with the LAGB. Following such a criterion, now we have two nanograins with twins; their mutual misorientation ( φ ) is shown in the inset of Fig. 6 . Once θ i ≤ θ c ( i =1, 2 or 3), G1 and G2 would coalesce into a large grain with the LAGB. Here θ i is the smallest rotation angle and the method to get θ i has been described above. We calculate the possible ϕ between G1 and G2 suitable for θ i ≤ θ c through the rotation around four typical low-index symmetric axes < hkl > in the fcc crystal, respectively, as shown in Fig. 6 . We find that there is a large possibility for the present mechanism to occur in G1 / G2 with ϕ < hkl >, especially for ϕ <110> ( ϕ =0–10°, 29–48.9°, 60.6–80.5°, 99.5–119.4°, 131.1–151° and 170–180°) and ϕ <111> ( ϕ =0–10°, 50–70°, 110–130° and 170–180°). Obviously, our experimental observations ( Table 2 ) are well consistent with the calculations, as shown by data points in Fig. 6 , that is, G3/G4 with ϕ =5.3° could coalesce through twin formation, while G5 / G3 with ϕ =87.2° and G5 / G4 with 82.2° still remained intact without any evident grain growth. 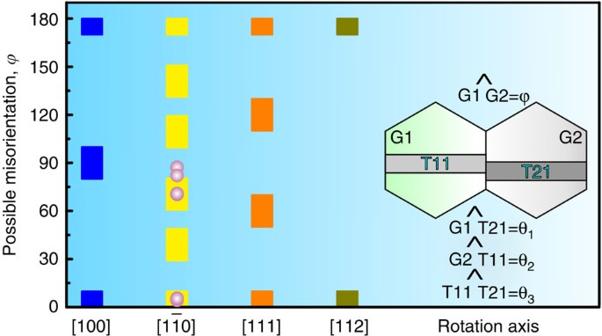Figure 6: Possibility for nanotwin-assisted grain coalescence. Possible misorientation angle (ϕ) suitable for nanograinsG1andG2coalescence induced by the present nanotwin-assisted mechanism under different rotation axes <hkl>. The inset shows all the misorientation angles among grains and twins. Figure 6: Possibility for nanotwin-assisted grain coalescence. Possible misorientation angle ( ϕ ) suitable for nanograins G1 and G2 coalescence induced by the present nanotwin-assisted mechanism under different rotation axes < hkl >. The inset shows all the misorientation angles among grains and twins. Full size image Table 2 Mutual misorientation angles among grains and twins. Full size table Once the grain coarsens, the perfect dislocation activity gradually tends to be effective and the GB motion velocity decreases. Hence, although the orientation relationship between the coarsened grain and the next neighbouring grain may be satisfied, the nanotwin-assisted mechanism may not have the grains to grow so large that fatigue extrusions/intrusions are able to form, as observed in ultrafine grains produced by severe plastic deformation [46] . In the ultrafine grains with highly stored deformation energy, the thermally activated dynamic recovery resulted in grain coarsening and subsequent cyclic softening [2] , while the limited grain coarsening in the present nano-grained films led to the fact that the initiation of fatigue cracks is still rather difficult in these coarsened grains less than 100 nm [34] . Furthermore, such nanotwin-assisted grain growth may effectively dissipate some amount of cyclic plasticity, and thus partially contribute to enhanced fatigue properties of the 20-nm-thick gold films compared to that of 900-nm-thick ones, as shown in Fig. 7 . Although there are almost no reports on fatigue properties of bulk polycrystalline gold, the comparison of the nc gold films to bulk polycrystalline copper [47] , micron-thick copper films [48] , [49] and submicron-thick copper films on polyimide substrates [48] , [49] demonstrates that the nc gold films is of much higher fatigue strength than that of the submicron-scale copper films and the bulk copper (see Fig. 7 ), indirectly revealing that fatigue properties of the nc gold films are evidently enhanced compared with the bulk ones. In addition to the potential contribution from high strengths of the nanograins and the nanotwins, this improvement in fatigue properties may also be closely associated with the limited coarsening of nanograins, which is assisted by cyclic loading-sustained nanotwin formation. 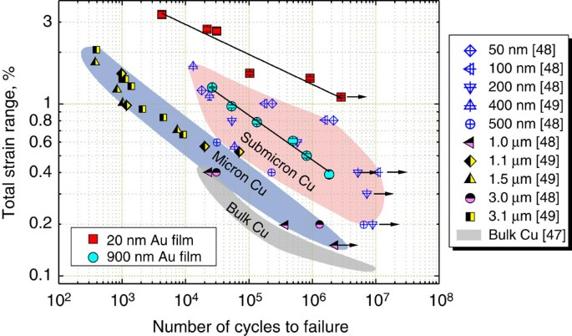Figure 7: Comparison of fatigue life. Fatigue strength of 20-nm-thick gold films is evidently higher than that of the 900-nm-thick ones. The fatigue strengths of the gold films were also compared with the datum of bulk polycrystalline copper, micron-thick copper films and submicron-thick copper films on polyimide substrates reported in the literature. Figure 7: Comparison of fatigue life. Fatigue strength of 20-nm-thick gold films is evidently higher than that of the 900-nm-thick ones. The fatigue strengths of the gold films were also compared with the datum of bulk polycrystalline copper, micron-thick copper films and submicron-thick copper films on polyimide substrates reported in the literature. Full size image In fact, Fang et al. [50] have recently shown that mechanically driven grain growth did play a key role in enhancing plasticity of gradient nc copper, unveiling the potential plasticity in the high-strength nc materials. We expect that such nanotwin-assisted grain growth mechanisms may validate only in the nanoscale regime where PDs have taken over as the main cyclic deformation way, but the proposed mechanism would be of considerable technological importance to the optimum design of GB stability through the concept of the limited coarsening of the nanograins assisted by nanotwins for high-performance nanostructured materials with both high strength and good fatigue resistance. Our findings reveal, in general, that the grain growth of the nano-grained gold films under cyclic loading is related to nanotwin formation, which plays a key role in changing local grain orientation and dissociating boundaries of nanograins. As a result, the grain growth can be assisted effectively. The proposed nanotwin-assisted grain growth mechanism and the theoretical calculation of crystallographic relationship among the neighbouring grains may provide a clue how to stabilize the nano-GBs, and even modulate cyclic plasticity of nc metals through the optimum design of the nano-GBs for the GB engineering. Sample preparation We deposited 20-nm-thick gold films (target purity: 99.99%) onto 125 μm-thick polyimide (Dupont Kapton) substrates using DC magnetron sputtering under ultra-high vacuum (10 −7 torr) conditions. Before deposition, the substrate was cleaned by sputtering Ar ions for ~5 min to remove the surface contamination and to improve the bond between the substrate and the film. Experimental methods Fatigue tests of the film samples with a gauge section of 13 mm in length and 3 mm in width were performed under load control at a frequency of 20 Hz and load ratio (the minimum load/the maximum load) of 0.1. To introduce fatigue damage in the sample, an initial load range (Δ P ) was applied to the film bonded to the elastic polyimide substrate for a fixed 10 6 cycle-testing. Then, Δ P was not increased successively until the discernable cracks appeared in the film within 10 6 cycles. The critical Δ P needed to generate fatigue damage within 10 6 cycles was determined to be 16.0 N, which corresponds to the total strain range of 1.41%. The samples for observations on fatigue damage behaviour ( Figs 1 , 2 , 3 and Supplementary Figs 1–3 ) were conducted by this method. In order to evaluate fatigue life, fatigue tests of the gold film samples with a gauge section of 10 mm in length and 3 mm in width were performed under load control at a frequency of 20 Hz for high cycle regime (>10 5 cycles) and 1 Hz for low cycle regime. Load ratio is also 0.1. A real-time electrical resistance ( R ) of the film was measured during cyclic loading using a digital multimeter (Agilent 34410A) with a resolution of 10 −3 Ω. An increase in Δ R / R 0 (Δ R = R − R 0 and R 0 is the initial electrical resistance before fatigue testing) is considered to be associated with the nucleation and propagation of cracks in the film, which was confirmed by the postmortem SEM observations. To determine the critical Δ R / R 0 corresponding to the onset of fatigue cracking, we conducted a series of the postmortem SEM observations at different Δ R / R 0 (see Supplementary Fig. S5 ). Thus, the number of cycles to failure is determined to be the fatigue cycles at which Δ R / R 0 increases to 10%, where the macrocrack starts to propagate, resulting in the failure of the film. Similar definitions of the fatigue life were adopted in former reports [51] , [52] , [53] . Characterization The samples for HRTEM and TEM investigations were ground mechanically to ~30 μm in thickness, and then further thinned by ion milling on a precision ion polishing system (Gatan 691) at −100 °C. A field emission gun SEM (Zeiss Supra 35) and a field emission gun TEM (FEI Tecnai F20) were used to observe the gold films. HRTEM observations were operated at 200 kV and its point resolution is ~0.21 nm. X-ray diffraction θ –2 θ scans were recorded on a Rigaku X-ray diffractometer D/MAX–2500/PC equipped with Cu Kα radiation (56 kV, 182 mA). How to cite this article: Luo, X.-M. et al. Nanotwin-assisted grain growth in nanocrystalline gold films under cyclic loading. Nat. Commun. 5:3021 doi: 10.1038/ncomms4021 (2014).